Synergistic Pd/Cu-catalyzed enantioselective Csp2–F bond alkylation of fluoro-1,3-dienes with aldimine esters Due to high bond dissociation energies of Csp 2 –F bonds, using fluorinated compounds in Csp 2 –Csp 3 cross-coupling is difficult. Here the authors report a protocol for enantioselective Csp 2 –Csp 3 coupling of dienyl fluorides with aldimine esters, enabled by synergistic copper and palladium catalysis. This reaction represents the first example of asymmetric Csp 2 –Csp 3 cross-coupling involving an inert Csp 2 –F bond and provides expeditious access to chiral α-alkenyl α-amino acids with high enantioselectivity. Control experiments suggest that the Csp 2 –F bond activation occurs through a pathway involving PdH migratory insertion and subsequent allylic defluorination, rather than by direct oxidative addition of the Csp 2 –F bond to Pd(0). The detailed mechanism is further investigated by DFT calculation and the enantioselectivity is rationalized. Transition-metal-catalyzed enantioselective cross-coupling reactions between Csp 2 –X compounds (X = halogen) and enolizable carbonyl compounds are commonly used transformations for asymmetric construction Csp 2 –Csp 3 bonds [1] , [2] , [3] , [4] , [5] , [6] , [7] . Many successful examples of this method have been reported, including pioneering work by the research groups of Ma [1] , Hartwig [2] , and Buchwald [3] , [6] , who used chiral-ligand-bearing transition metals such as Cu and Pd to achieve enantiocontrol (Fig. 1a ). These reactions initiated with oxidative addition of Csp 2 –X bond to the Pd(0) or Cu(I), followed by ligand exchange and reductive elimination to form the Csp 2 –Csp 3 bond. Halogenated compounds with Csp 2 –I, Csp 2 –Br, and even Csp 2 –Cl bonds are suitable reaction substrates. However, because Csp 2 –F bonds have high energies (120–129 kcal/mol for olefinic C–F bonds), fluorinated compounds have rarely been used as coupling partners [8] , [9] , [10] , [11] , [12] , [13] , [14] , [15] . Fig. 1: Transition-metal-catalyzed asymmetric Csp 2 –Csp 3 cross-coupling reactions. a Enantioselective Csp 2 –Csp 3 cross-coupling of Csp 2 –I (Br, Cl) Bonds. b C–F bond Activation by Nu-M Insertion/β-fluorine elimination. c This work: C–F bond activation by Pd-H insertion/allylic defluorination for Csp 2 –Csp 3 cross-coupling. Full size image Recently, C–F activation has been an important research topic in synthetic organic chemistry [16] , [17] , [18] , [19] , [20] . One of the most successful strategies in this area is using transition-metal-mediated or -catalyzed metal-Nu insertion/β–F elimination process [21] . Trifluoro-, difluoroalkenes have been intensively investigated for this purpose during the past few years [22] , [23] , [24] , [25] , [26] , [27] , [28] , [29] , [30] ; however, monofluoroalkenes are rarely explored class of compounds for similar C–F activation reactions (Fig. 1b ). Moreover, despite those achievements in defluorinative carbon–carbon and carbon–heteroatom bond formation, enantioselective variants have seldom been realized. We envisioned that if an ingenious insertion/β–F elimination mechanism was designed together with a suitable chiral induction strategy, the aforementioned challenged defluorinative Csp 2 –Csp 3 coupling might be achieved. In this work, we report a Cu/Pd cooperative system [31] for enantioselective Csp 2 –Csp 3 cross-coupling between dienyl fluorides and aldimine esters (Fig. 1c ). Experimental and computational studies revealed that this reaction involved a unique Pd-H insertion/allylic defluorination process. This work not only represents the first example of enantioselective defluorinative Csp 2 –Csp 3 coupling but also provides a highly efficient catalytic method to prepare chiral α-alkenyl α-amino acids (α-AAs), which are important synthetic targets [32] , [33] , [34] , [35] , [36] because of their potential biochemical and pharmacological activities [37] . Reaction development Our studies begin with investigating the reaction of dienyl fluoride E - 1a with aldimine ester [38] , [39] , [40] 2a to generate α-alkenyl, α-methyl α-AA 3aa . 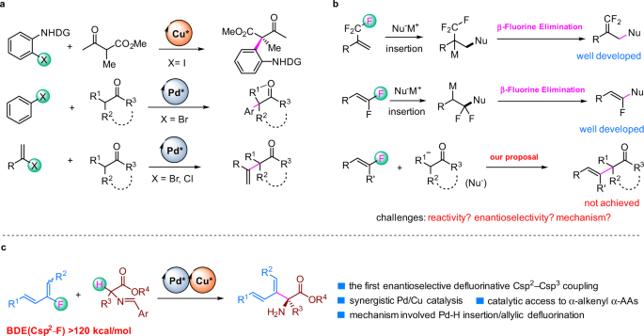Fig. 1: Transition-metal-catalyzed asymmetric Csp2–Csp3cross-coupling reactions. aEnantioselective Csp2–Csp3cross-coupling of Csp2–I (Br, Cl) Bonds.bC–F bond Activation by Nu-M Insertion/β-fluorine elimination.cThis work: C–F bond activation by Pd-H insertion/allylic defluorination for Csp2–Csp3cross-coupling. Using the stereocontrol exhibited by Cu-azomethine ylides in two-metal catalytic systems [41] , [42] , [43] , we designed a synergistic Pd/Cu catalyst system [44] , [45] , [46] , [47] , [48] , [49] , [50] , [51] , [52] , [53] , [54] , [55] for controlling the stereochemistry of the newly formed chiral center by means of an appropriate combination of ligands on the two metals during the coupling step (Table 1 ). First, we tested Phosferrox Cu complex L1-Cu with Pd catalysts bearing a bisphosphine ligand (dppe, dppp, Xantphos, or DPEphos; L4-Pd – L7-Pd , respectively) and found that none of these combinations catalyzed the desired reaction (entries 1–4). In contrast, BINAP-ligated catalyst L8-Pd afforded 3aa in 53% yield with 96% ee (entry 5). SEGPHOS- and Biphep-derived catalysts ( L9-Pd – L11-Pd , entries 6–8) were also examined, and L11-Pd gave the best yield of the product. Subsequent tests of L11-Pd in combination with other Cu catalysts ( L2-Cu and L3-Cu , entries 9 and 10) revealed that L11-Pd / L3-Cu gave the best results (86% yield, 99% ee). A slight decrease in enantioselectivity was observed when the opposite enantiomer of the Pd catalyst ( ent -L11-Pd ) was used together with L3-Cu (entry 11). This result implies the enantioselectivity was mainly controlled by the chiral Cu catalyst but the mismatched chirality between the two catalysts was slightly deleterious to the enantiocontrol. Table 1 Optimization of catalyst system for the cross-coupling reaction. Full size table Substrate scope Having developed an effective dual-metal catalyst system, we investigated the substrate scope of the reaction, starting with dienyl fluorides 1 bearing various R 1 and R 2 substituents (Fig. 2 ). Phenyl rings with a methyl group ( 3ba , 3ca ), a fluorine atom ( 3da – 3fa ), a chlorine atom ( 3ga ), a trifluoromethyl group ( 3 ha ), or a methoxy group ( 3ia ) were well tolerated, regardless of the location of the substituent, affording the corresponding coupling products in 71–87% yields with enantioselectivities exceeding 98% ee. Replacing the phenyl ring with a different aromatic ring—naphthyl ( 3ja ), furyl ( 3ka ), thiophenyl ( 3la ), or indolyl ( 3ma )—had little influence on the reaction outcome, the corresponding α-alkenyl, α-alkyl α-AAs were obtained with excellent enantioselectivities. An alkyl-substituted substrate (R 1 = cyclohexyl) furnished 3na in 63% yield, albeit with a reduced ee (94%). Even though allylic ethers are commonly sensitive to Pd owing to the possibility of C–O bond cleavage, a substrate with an allylic BnO ether moiety was well tolerated in this reaction system, giving 3oa in 60% yield with 99% ee. A 1,4-disubstituted dienyl fluoride (R 1 = Ph, R 2 = Me) was also investigated, which afforded the desired product 3pa in 50% yield with >99% ee. To determine the stereochemistry of the product, we converted 3aa to its p -toluenesulfonamide derivative and confirmed its structure by means of X-ray crystallographic analysis, which allowed us to assign the absolute configuration as 2 S . Fig. 2: Substrate scope with respect to the dienyl fluorides. Reaction conditions: (i) 1a (0.4 mmol), 2a (0.2 mmol), L11-Pd (4 mol%) , L3-Cu (5 mol%), Et 3 N (200 mol%), THF (0.5 mL), 30 °C, 24 h; (ii) citric acid (10 wt%, 4 mL). Isolated yields are provided. The ee values were determined by HPLC on a column with a chiral stationary phase. a L11-Pd (8 mol%), L3-Cu (10 mol%), THF (0.2 mL), 40 °C, 120 h. Full size image Next, we probed the scope of aldimine esters substrate (Fig. 3 ). When R 4 was methyl, R 3 could be Et ( 3ab ), n Bu ( 3ac ), or phenylethyl ( 3ad ). Heteroatom-tethered alkyl chains were also well-tolerated, as indicated by the formation of coupling products 3ae – 3ag in moderate to good yields with good enantioselectivities. In addition, we investigated compounds with various alkyl R 4 groups ( 3ah – 3aj ), revealing that the reaction was not sensitive to the steric bulk of the ester. An aldimine ester derived from glutamic acid also reacted smoothly but gave lactam 3ak in 58% yield with 92% ee, as a result of cyclization during the acidic workup. α-Amino-γ-butyrolactone derived imine underwent reaction with 1a to give 3al in moderate yield. In addition to aldimine ester, cyclic ketimine ester and oxazoline ester were also compatible reaction partners. As shown in the formation of 3am and 3an , both the yields and enantioselectivities were well maintained for these types of nucleophiles. Phenylalanine derived aldimine ester 2o failed to undergo this transformation due to the steric bulk, and substrate 2p bearing allyl group only gave complexed products, probably because the isomerization of the terminal olefin moiety. Fig. 3: Substrate scope with respect to the aldimine esters. Reaction conditions: (i) 1a (0.4 mmol), 2a (0.2 mmol), L11-Pd (4 mol%), L3-Cu (5 mol%), Et 3 N (200 mol%), THF (0.5 mL), 30 °C, 48 h; (ii) citric acid (10 wt%, 4 mL). Isolated yields are provided. The ee values were determined by HPLC on a column with a chiral stationary phase. Full size image Synthetic application The reaction was scaled up to more than one mmol scale with a reduced catalyst loading [ L11-Pd (2 mol%) and L3-Cu (2.5 mol%)] and the yield and enantioselectivity were well maintained (Fig. 4a ). To demonstrate the utility of the reaction, the coupling products were transformed to other chiral scaffolds. Protection ( S )- 3aa with p -tolylsulfonyl group gave ( S )- 4aa , and the latter was treatment with NBS/Na 2 CO 3 in acetonitrile to elaborate the bromoamination product 5aa in 75% yield (Fig. 4b ). The internal alkene moiety of ( S )- 4aa could be selectively cleaved with K 2 Os(OH) 4 /NMO, followed by NaIO 4 , affording aldehyde ( S )- 6aa in 86% yield (Fig. 4c ). Moreover, protection the amine of ( S )- 3oa with benzoyl group gave ( S )- 4oa , which was further subjected to sequential dihydroxylation/lactonization conditions to furnish densely functionalized lactone 5oa with good diastereoselectivity (Fig. 4d ). Fig. 4: Synthetic application. a Scale-up reaction at lower catalyst loading. b Intramolecular bromoamination reaction. c Selective cleavage of the internal alkene. d Dihydroxylation/lactonization reaction. Full size image Mechanistic studies To gain insight into the mechanism, we carried out some control experiments. We found that reactions of both >20:1 and 1:1 E / Z- 1a gave >20:1 E / Z- 3aa with essentially identical yields and ee values (Fig. 5a ). On the other hand, when 1a with the E/Z ratio of 1:1.1 was subjected to the reaction, the absolute amount of the Z - 1a and E - 1a was monitored (Fig. 5b ). Interestingly, the concentration of Z - 1a and E - 1a are both decreased during the reaction; however, the E - 1a has a faster consumption rate than Z - 1a did. Most importantly, an inflection point appeared around 5 h in the E - 1a consumption curve. These results indicate a possibility that E - 1a preferentially reacted under the optimized conditions at the early stage, and Z - 1a gradually isomerized to E - 1a . In addition, when dienyl bromide 4a or dienyl chloride 4b was subjected to the reaction conditions, almost none of the coupling product ( 3aa ) was observed (Fig. 5c ). Consequently, we reasoned that direct oxidative addition of the Csp 2 –F bond to Pd(0) was probably not involved in the reaction pathway [56] , [57] . Finally, the reaction between 1a and deuterium-labeled 2a resulted in the incorporation of a total 30% of the deuterium at the terminal carbon of the double bond in the coupling product (Fig. 5d ). As a result, we speculated that a Pd–D insertion process might be involved in the reaction, which would lead to deuterium enriching at the terminus of the alkenes [58] . Fig. 5: Control experiments. a Relationship between the ratio of Z / E - 1a and ratio of Z / E - 3aa . b The absolute amount the Z- 1a and E - 1a during the reaction. c Reaction of dienyl bromide 4a or dienyl chloride 4b under the standard conditions. d Deuterium atom scramble experiment. Full size image Based on the above-described results, as well as our previous studies [59] , [60] on synergistic Pd/Cu-catalyzed coupling reactions of aldimine esters with unsaturated compounds, we proposed that this coupling reaction proceeds based on a mechanism involving the Cu and PdH cycles shown in Fig. 6 . In the Cu catalytic cycle, Cu acts as a Lewis acid to activate aldimine ester 2a to form metallated azomethine ylide II , which serves as a nucleophile in the coupling reaction. Allylation of II with pre-palladium catalyst L11-Pd forms the L11-Pd (0), which then undergoes oxidative addition with Et 3 NH + to generate the PdH catalyst (Fig. 6a ). In the PdH catalytic cycle (Fig. 6b ), PdH migratory insertion into the C = C bond of the vinyl fluoride moiety of E - 1a generates fluorinated Pd-allyl III [61] , [62] , [63] , [64] . An allylic substitution reaction between III and metallated azomethine ylide II affords Pd intermediate IV and regenerates the Cu catalyst. Intermediate IV undergoes rapid allylic defluorination, giving allyl-Pd V , which is converted to VI via β-H elimination. Product 3aa dissociates from VI , and the PdH regenerated [65] , [66] , [67] . For Z - 1a , the anti-anti η 3 -Pd-allyl VII is generated after PdH migratory insertion, which equilibrates to thermodynamically more stable syn-anti η 3 -Pd-allyl III through η 3 - η 1 - η 3 isomerization (Fig. 6c ). Therefore Z - 1a would then undertake the same catalytic cycle to form the same E -type product 3aa . This proposed mechanism was highly consistent with the controlled experiments in Fig. 3 . Moreover, we observed a [M + H] + signal at 252.1393 in the HRMS spectrum of the reaction mixtures. This result indicates the formation of IX , which comes from the dissociation of Pd(0) from intermediate IV (Fig. 6d ). Fig. 6: Proposed mechanism. a Initial generation of PdH catalyst from the precatalyst L11-Pd . b Proposed catalytic cycle. c Isomerization of anti - anti π-allyl-Pd to syn - anti π-allyl-Pd. d HRMS detection of [M + H] + for Intermediate IX. The ligands were omitted for clarity. Full size image Computational studies To further understand the mechanism, we performed DFT calculation to investigate the energy profile of this reaction. Stoichiometric reaction of L3-Cu and substrate 2a with DBU, only one isomeric Cu-azomethine ylide was formed, as indicated by a single 31 P NMR signal at −16.09 (Fig. 7 ). The structures of Cu-azomethine ylide featuring a ( R )- or ( S )- metal chirality were calculated and we found the former is 2.9 kcal/mol stable than the latter. Therefore, we rationalized that Cu( R )-Nu rather than Cu( S )-Nu was the form for nucleophile and therefore its structure was adopted for the remaining DFT calculation (Fig. 8 ). Fig. 7: Determination of the structure for the Cu-azomethine ylide. a Observation of the Cu-zaomethine ylide by 31 P NMR. b Energy comparison of Cu( R )-Nu and Cu( S )-Nu. Full size image Fig. 8: Energy profile for the proposed mechanism. Calculations were carried out at the M06-2x(SMD)/def2-TZVP//B3LYP-D3BJ/6-31 g(d)/Lanl2dz level of theory. Full size image As proposed in Fig. 8 , the PdH was initially formed via oxidative protonation of Pd(0) with Et 3 NH + . The transition state for this step was located as TS-1 , which has an energy barrier of 15.0 kcal/mol. After being coordinated by substrate 2a , the resulting intermediate Int-2 occurs migratory insertion of the Pd–H bond into the terminal olefin moiety to afford π-allyl-Pd species Int-4 . The energy barrier for this step is only 1.1 kcal/mol; however, the reserved β–H elimination step requires activation energy of 29.7 kcal/mol ( Int-4 → TS-3 → Int-2 ). Therefore, the Pd–H migratory insertion is not a reversible process. The resulting Int-4 accepts nucleophilic attach from the si -face of the metallated azomethine ylide Cu-Nu, to give C–C bond formation intermediate Int-6 . Dissociation of LCu from Int-6 affords species Int-7 , which then undergoes allylic defluorination. The direct nucleophilic displacement/ionization mechanism for the defluorination transition state ( TS-8A ) has a high energy barrier of 28.0 kcal/mol. But a Et 3 NH + mediated process, of which the transition state was located as TS-8B , only requires an activation barrier of 12.2 kcal/mol. The resulting Int-9 then occurs β–H elimination step via TS-10 with an energy barrier of 27.5 kcal/mol to elaborate product ( 2 S )- 3aa and regenerates the PdH catalyst. To elucidate the enantioselectivity, the approach from the re -face of Cu-Nu during the C–C bond formation was also calculated and the transition state is identified as TS-5-II (Fig. 9a ). 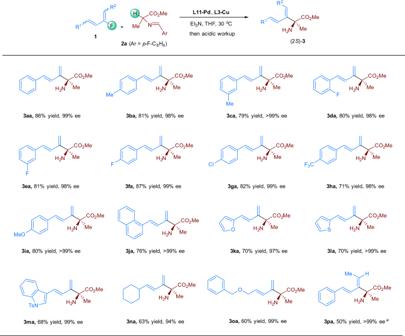Fig. 2: Substrate scope with respect to the dienyl fluorides. Reaction conditions: (i)1a(0.4 mmol),2a(0.2 mmol),L11-Pd(4 mol%), L3-Cu(5 mol%), Et3N (200 mol%), THF (0.5 mL), 30 °C, 24 h; (ii) citric acid (10 wt%, 4 mL). Isolated yields are provided. The ee values were determined by HPLC on a column with a chiral stationary phase.aL11-Pd(8 mol%),L3-Cu(10 mol%), THF (0.2 mL), 40 °C, 120 h. Comparing the energies of TS-5 and TS-5-II , the latter is disfavored over the former by 5.0 kcal/mol, which is in agreement with the experimental result that ( 2 S )- 3aa is formed with 99% ee. In the transition state structure TS-5-II , the oxazoline ring group on the phosferrox ligand has a very short distance away from t- Bu groups of DTB-Biphep and which leads to significant steric interaction between the two ligands (Fig. 9b ). This repulsive interaction likely contributes to the higher energy observed for this competing transition state. 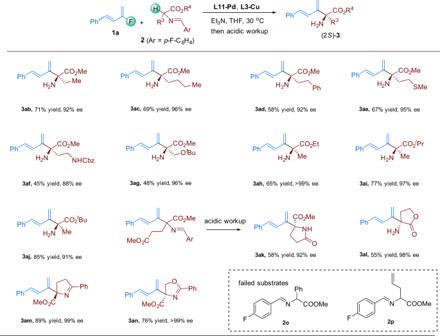Fig. 3: Substrate scope with respect to the aldimine esters. Reaction conditions: (i)1a(0.4 mmol),2a(0.2 mmol),L11-Pd(4 mol%),L3-Cu(5 mol%), Et3N (200 mol%), THF (0.5 mL), 30 °C, 48 h; (ii) citric acid (10 wt%, 4 mL). Isolated yields are provided. The ee values were determined by HPLC on a column with a chiral stationary phase. In contrast, in the transition state structure TS-5 , the electrophile approaches from the si -face of Cu-Nu which avoids the steric repulsion between the oxazoline ring and t- Bu groups. Moreover, an attractive C–H ∙ ∙ ∙ Ar interaction is observed in TS-5 , which also contributes to a lower energy (Fig. 9c ). Fig. 9: Rationalization of the enantioselectivity. a Comparison of Transition states TS-5 and TS-5-II . b Steric interaction between the oxazoline ring and t -Bu group in TS-5-II . c Attractive C–H ⋯ Ar interaction in TS-5 . 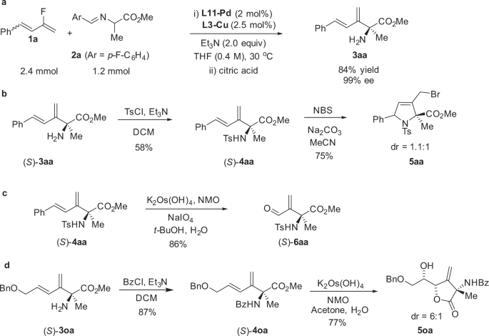Fig. 4: Synthetic application. aScale-up reaction at lower catalyst loading.bIntramolecular bromoamination reaction.cSelective cleavage of the internal alkene.dDihydroxylation/lactonization reaction. Full size image In summary, the first enantioselective defluorinative Csp 2 –Csp 3 cross-coupling was achieved by means of synergistic Cu/Pd-catalyzed asymmetric coupling between aldimine esters and dienyl fluorides. This reaction has a wide substrate scope and shows good to excellent enantioselectivities and it provide an efficient catalytic method for preparing chiral α-vinyl, α-alkyl α-amino acid derivatives. Both experimental and computational studies revealed that the reaction is initiated by a PdH migratory insertion, which is followed by nucleophilic allylic substitution by a Cu-azomethine ylide to form the C–C bond. Then a Pd/Et 3 NH + -mediated allylic defluorination undergoes, subsequently followed by a β–H elimination to elaborate the coupling product and regenerate the PdH catalyst. General procedure for coupling of dienyl flurides and aldimine esters In glove box, Cu(MeCN) 4 PF 6 (3.7 mg, 0.01 mmol, 5 mol%) and chiral ligand ( S,S p )- L3 (5.3 mg, 0.011 mmol, 5.5 mol%) were dissolved in dry THF (0.4 M, 0.5 mL) and stirred at room temperature for 0.5 h. To the solution, substrate aldimine esters 2 (0.2 mmol), Et 3 N (0.4 mmol), dienes 1 (0.4 mmol) and palladium catalyst L11-Pd (10.1 mg, 0.008 mmol, 4 mol%) were added sequentially. The reaction mixture was stirred at 30 °C for 24 h. To the reaction mixture was added citric acid solution (4 mL, 10 wt%) and the mixture was stirred for 2 h. The mixture was neutralized with solid K 2 CO 3 and extracted with EtOAc (10 mL × 3). 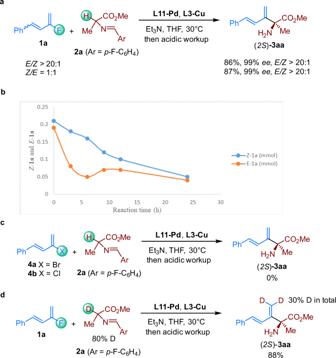Fig. 5: Control experiments. aRelationship between the ratio ofZ/E-1aand ratio ofZ/E-3aa.bThe absolute amount theZ-1aandE-1aduring the reaction.cReaction of dienyl bromide4aor dienyl chloride4bunder the standard conditions.dDeuterium atom scramble experiment. The combined extracts were dried over MgSO 4 and concentrated in vacuo to afford a residue. 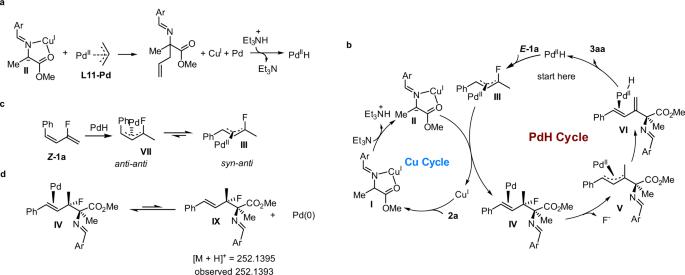Fig. 6: Proposed mechanism. aInitial generation of PdH catalyst from the precatalystL11-Pd.bProposed catalytic cycle.cIsomerization ofanti-antiπ-allyl-Pd tosyn-antiπ-allyl-Pd.dHRMS detection of [M + H]+for Intermediate IX. The ligands were omitted for clarity. 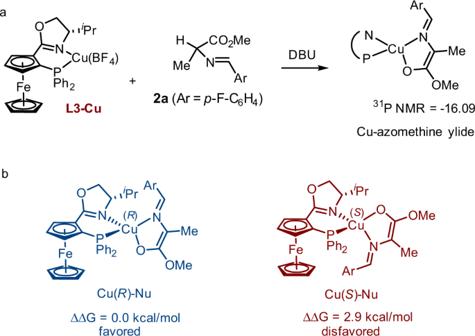Fig. 7: Determination of the structure for the Cu-azomethine ylide. aObservation of the Cu-zaomethine ylide by31P NMR.bEnergy comparison of Cu(R)-Nu and Cu(S)-Nu. 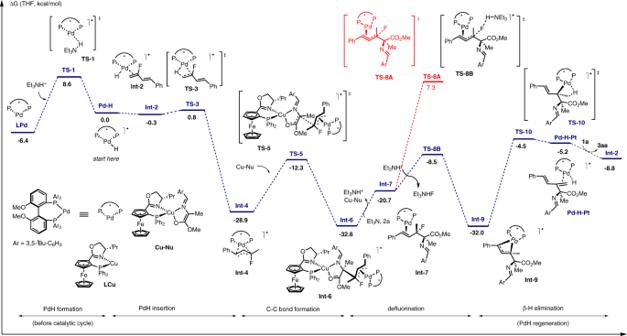Fig. 8: Energy profile for the proposed mechanism. Calculations were carried out at the M06-2x(SMD)/def2-TZVP//B3LYP-D3BJ/6-31 g(d)/Lanl2dz level of theory. 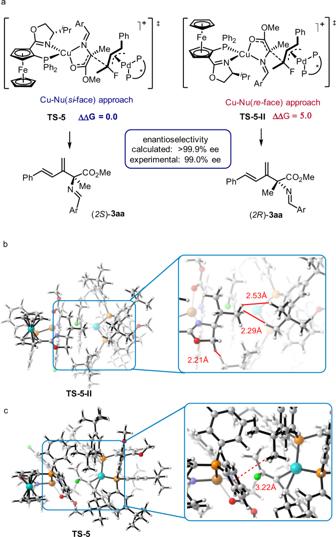Fig. 9: Rationalization of the enantioselectivity. aComparison of Transition statesTS-5andTS-5-II.bSteric interaction between the oxazoline ring andt-Bu group inTS-5-II.cAttractive C–H⋯Ar interaction inTS-5. The residue was then purified by SiO 2 column chromatography to give the desired product.